Localized states in advanced dielectrics from the vantage of spin- and symmetry-polarized tunnelling across MgO Research on advanced materials such as multiferroic perovskites underscores promising applications, yet studies on these materials rarely address the impact of defects on the nominally expected materials property. Here, we revisit the comparatively simple oxide MgO as the model material system for spin-polarized solid-state tunnelling studies. We present a defect-mediated tunnelling potential landscape of localized states owing to explicitly identified defect species, against which we examine the bias and temperature dependence of magnetotransport. By mixing symmetry-resolved transport channels, a localized state may alter the effective barrier height for symmetry-resolved charge carriers, such that tunnelling magnetoresistance decreases most with increasing temperature when that state is addressed electrically. Thermal excitation promotes an occupancy switchover from the ground to the excited state of a defect, which impacts these magnetotransport characteristics. We thus resolve contradictions between experiment and theory in this otherwise canonical spintronics system, and propose a new perspective on defects in dielectrics. Today’s information technology society is predicated upon the mastery of growing high-quality, archetypical semiconductors such as Si and GaAs within ever more refined heterostructures. This notably involved an explicit, 40-year study of, and control over, defects within these key historical semiconductors. Against this backdrop of painstaking, difficult and thus meticulous materials defect research, a different materials research paradigm is emerging. With societal goals ranging from enhanced, multilevel memories to artificial synapses to energy harvesting, this research paradigm aims to rapidly deploy the intrinsic properties of novel, advanced materials within device heterostructures with enhanced functionalities. For instance, multiferroics such as GaFeO 3 (ref. 1 ) intertwine the material’s internal magnetic and electric degrees of freedom to promote a path towards multilevel memories. Also, a memristive device based on ferroelectricity was reported with applications, for instance, as hardware-oriented artificial synapses [2] . Thus, within the present materials research paradigm, both the fast pace of today’s research and the sheer number of materials candidates mostly preclude the possibility to meticulously study structural defects within these advanced materials. This impedes an assessment of the impact that such defects may have on the nominally expected materials property. For instance, magnetic tunnel junctions (MTJs) that comprise a ferroelectric [3] or multiferroic [4] barrier yield devices with four addressable states, yet the same result may be achieved with a simple paraelectric barrier with altered stoichiometry [5] , [6] , [7] , [8] . Furthermore, at the nanoscale, defects shall strongly affect a dielectric material’s effective properties, including the intrinsic property that prompted initial research interest in the material. This impact of defects on the dielectric material’s nominally expected properties has, for instance, led to controversy in the field of oxide-based dilute magnetic semiconductors [9] . It has also proven useful to understand the properties of two-dimensional electron gases at the interfaces between correlated oxides [10] , [11] . In the present work, we focus on the comparatively simple oxide MgO. Epitaxial or textured MgO-based MTJs are deemed to constitute a canonical example of spin-polarized solid-state tunnelling [12] , with applications ranging from read-heads of hard disk drives [13] to non-volatile random access memory [14] to magnetic sensors [15] or spin-torque nano-oscillators [16] . Yet tunnelling magnetoresistance ratios (TMRs) remain one order of magnitude below those predicted [17] . The impact of intrinsic effects such as magnon and phonon generation on TMR has been documented [18] , [19] . On the other hand, the impact of structural defects in MgO on tunnelling is only emerging in this otherwise widely studied, canonical spintronic system [20] , [21] , [22] , [23] , [24] , [25] , [26] . Indeed, defects have been qualitatively suspected of accounting for much lower tunnelling barrier heights than expected [12] , [27] . Defects are thus generically considered to hinder magnetotransport [28] . This has spurred efforts to control the density of oxygen vacancies during MgO growth [27] , although a more recent theory suggests that spatially close oxygen vacancies, or even paired oxygen vacancies known as M centres, lead to symmetry-conserving transport [25] . However, without knowing of precisely which defect species is responsible for altering magnetotransport in a given MTJ, it is difficult to understand, let alone control, the impact of defects on magnetotransport. This immature state-of-the-art is all the more surprising considering that defects within MgO-based MTJs may be magnetic [29] , [30] , [31] , and are thought to underscore advanced device functionalities such as memristive effects [22] , [32] , [33] , which may be likened to the operation of a synapse-neuron pathway [34] . As an example of utilizing defects in advanced oxides, we aim to recast the foundation of spin-polarized solid-state tunnelling, within the canonical Fe/MgO system, on a more solid footing that explicitly accounts for how a precise defect species impacts solid-state tunnelling across MgO. In simple terms, this foundation rests upon a substantially lower tunnelling barrier height φ across MgO for electrons with Δ 1 electronic symmetry compared with Δ 5 electrons [35] , [36] , [37] . It is in turn the strong spin polarization of Δ 1 electrons at the Fermi level E F in bcc-oriented Fe, Co, FeCo and FeCoB alloys that leads to predicted TMR values of 10,000%. Experimentally, beyond initial experiments that confirm this band structure mechanism of spin-polarized solid-state tunnelling [38] , [39] , [40] , [41] , [42] , TMR values that reach 1,100% (600%) at low (room) temperature [43] confirm the broad outlines of this theoretical backdrop. Nevertheless, several aspects of this apparently clear foundation remain puzzling. Why is the highest experimental TMR [43] one order of magnitude lower than that predicted [35] , [36] ? Why does the TMR signal decrease so much with increasing temperature? The answer lies in resolving a third contradiction. 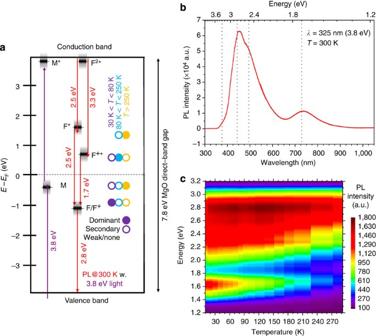Figure 1: Oxygen vacancies in MgO. (a) Schematic diagram of the energy positions of oxygen vacancies in the MgO barrier49,50,54,69. SeeSupplementary Note 1for further details. PL processes resulting from 3.8 eV optical excitation are also represented. A legend depicts for each localized state the robustness of thermal addressing within specific T ranges. (b) Typical PL spectrum atT=300 K and (c) temperature dependence of the PL spectrum from MgO(2.5 nm) tunnel barriers collected after excitation with 3.8 eV light. Data inbforλ<350 nm has been zeroed. As seen in Table 1 , deduced experimental barriers heights φ for the top performing MTJs may reach a mere 0.4 eV, rather than the 3.9 eV expected considering the 7.8 eV band gap [37] and a MTJ Fermi level pegged to the charge-neutrality level at the band gap centre [44] . In addition, experiments reveal little difference between the values φ P and φ AP measured in the parallel (P) and antiparallel (AP) configurations of ferromagnetic electrode magnetizations. For instance, MTJs presented in this paper yield [45] =0.62 eV and =0.5 eV at room temperature and a TMR of ~100% at 10 mV applied bias [46] . These values are typical of results reported by certain members of the community (see Table 1 ). This is puzzling because tunnelling in the P(AP) states, and the ensuing large TMR, is understood to reflect dominant Δ 1 (Δ 5 ) transport [12] , [35] , yet φ (Δ 1 ) is theoretically quite smaller than φ (Δ 5 ), both in the bulk [37] and in the tunnel barriers of MTJs [35] , [36] . In other words, despite rather similar barrier heights for Δ 1 and Δ 5 electrons (or even φ (Δ 1 )> φ (Δ 5 ) ), which are both much lower than expected, large values of TMR are observed. Table 1 Spread of reported barrier heights in MgO MTJs. Full size table In the following, we resolve these apparent contradictions by considering the impact of defects on solid-state tunnelling. Indeed, these experimentally measured barrier heights emphasize those defined by localized defect states within the MgO band gap, and do not correctly weigh in tunnelling by holes(electrons) with respect to the valence(conduction) band edges as considered theoretically. This is how one can simultaneously obtain R P < R AP and φ P > φ AP . We find that thermal excitations promote an occupancy switchover from the ground to the excited state of a defect. This alters the effective, symmetry-dependent barrier heights, as well as the ensuing TMR when probed at a bias voltage that electrically addresses the relevant defect level. Defect-induced potential landscape of tunnelling across MgO While research on MgO defects remains immature compared with that for Si or GaAs, it is more advanced than that for other binary oxides such as TiO 2 (ref. 47 ) or the prototypical ternary oxide SrTiO 3 (ref. 48 ). In general terms, a defect defines an energetical potential well located in the dielectric band gap that contains neutral/charged ground states and corresponding excited states [49] . We present in Fig. 1a an energy diagram that summarizes literature [49] , [50] , [51] , [52] on the energy positions, within the MgO optical band gap of the ground and excited states (labelled *) of selected neutral and charged (labelled + ) structural defects. In general terms, oxygen vacancies, labelled F, may appear within the upper half of the band gap, while magnesium vacancies (not on the picture) appear closer to the valence band [53] (VB). This reflects the respective donor/acceptor roles of these two species of vacancies for the MgO dielectric. We also represent paired oxygen vacancies, or M centres [54] , and refer the reader to the Supplementary Note 1 and Supplementary Fig. 1 for further details. Figure 1: Oxygen vacancies in MgO. ( a ) Schematic diagram of the energy positions of oxygen vacancies in the MgO barrier [49] , [50] , [54] , [69] . See Supplementary Note 1 for further details. PL processes resulting from 3.8 eV optical excitation are also represented. A legend depicts for each localized state the robustness of thermal addressing within specific T ranges. ( b ) Typical PL spectrum at T =300 K and ( c ) temperature dependence of the PL spectrum from MgO(2.5 nm) tunnel barriers collected after excitation with 3.8 eV light. Data in b for λ <350 nm has been zeroed. Full size image To understand which defect species are present in the MgO tunnel barriers of our MTJ stacks, we have performed photoluminescence (PL) on FeCoB/MgO stacks that were also prepared under standard MTJ conditions (see Methods). Typical PL results, acquired at T =300 K and using 3.8 eV light to optically activate M centres, are shown in Fig. 1b . Comparing with the energy positions of oxygen vacancies shown in Fig. 1a , we broadly identify PL peaks in terms of transitions between the excited and ground states of F and F + centres. The small feature at 3.3 eV may also incorporate the PL resulting from M centres [52] , but owing to its negligible amplitude we conclude that the MgO barrier of our stack contains predominantly F/F + and F + * states. Figure 1c shows the temperature dependence of the PL spectrum on the MgO of our MTJs. The PL peak at 1.7 eV, which reflects a F + *→F + recombination, decreases markedly with increasing T within 4 K< T <300 K, while the PL peak at 2.8 eV, which reflects a F/F + to VB recombination, persists with increasing T . Taken together, and in agreement with the literature [52] , we infer that the F/F + population remains broadly constant within 4 K< T <300 K, while the F + * population increases markedly for T >80 K. Intrinsic and defect-mediated tunneling regimes Spin-polarized solid-state tunnelling spectroscopy on lithographically processed stacks [8] can reveal the junction electrodes’ electronic structure [12] , [55] , the junction’s symmetry-resolved barrier heights [37] and inelastic tunnelling phenomena [19] that includes hopping onto defect states [24] . We note that, since the Δ 1 complex loop, which spans the band gap and defines the wavefunction decay through tunnelling, is rather flat within at least ±1.1 eV about the band gap centre, both electron and hole tunnelling with respect to states above and below E F are considered [37] (rescaling the local density approximation (LDA)-derived 4.7 eV MgO band gap to its experimental value of 7.8 eV yields a flat Δ 1 band over 2.2 eV about the charge-neutrality level-pegged chemical potential [37] . F centres strongly alter the Δ 1 complex loop [28] , but we nevertheless observe hole tunnelling across the F centre.). Solid-state tunnelling across a dielectric containing structural defects shall occur with respect to these defects’ numerous energy levels. As such, models such as Simmons [56] or Brinkman [57] that consider only one barrier height fail to capture the complex tunnelling potential landscape mediated by defects. To circumvent this problem, we extend the Î method [37] , [45] , [58] by considering Î rel =( I T2 / I T1 )−1, where I T1 and I T2 are values of I obtained from I ( V ) measurements performed at consecutive temperatures T 2 > T 1 and d T = T 2 − T 1 . Peaks in Î may thus reveal the energy position relative to E F at which a feature (for example, band structure, defect levels) in the junction’s potential landscape state may, thanks to thermal excitation from T 1 to T 2 , provide an additional contribution to the current across the MTJ. As such, Î rel yields the impact of thermal excitation at a precise temperature. For a comparison of room-temperature results obtained this way with those yielded by the widely used Brinkman model [57] , please refer to Supplementary Note 2 ; Supplementary Figs 2–4 ; Supplementary Table 1 . In the first set of experiments performed on our MTJs using the Î rel method, we studied the transition from an intrinsic regime of magnetotransport to one mediated by tunnelling with respect to defect states. We present in Fig. 2 Î rel in the P and AP MTJ configurations for d T =10 K. We set aside the magnon generation region within E = E F ±0.1 eV. In a first regime for T <20 K, yields a peak at 0.8 eV that is not present in . We attribute this AP feature to Δ 1↑ electrons tunnelling into the bottom of the Δ 1↓ band of the electrode that collects the current [42] . Similarly, the minimum in at 1.35 eV is attributed to spectrally reaching the top of the Δ 1↑ band (without a reference to Co 0.4 Fe 0.4 B 0.2 band structure calculations, we average the Co and Fe energy levels from ref. 59 and neglect the impact of B. See p.154 of ref. 46 ). Above this voltage, despite additional thermal energy, the tunnelling rate across the junction is expected to decrease as no additional electrons states due to thermal broadening can collect the Δ 1 tunnelling current. 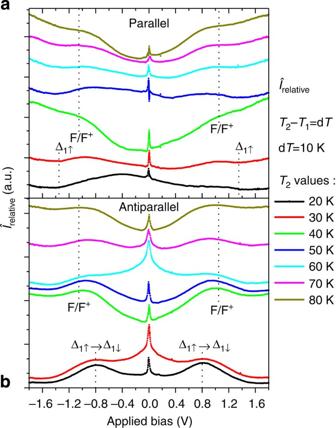Figure 2: Thermal switchover from intrinsic to defect-mediated tunnelling. Îrel(V,T) in the (a) P and (b) AP MTJ states within 9 K<T<80 K with dT=10 K. Consecutive curves are shifted upwards for clarity reasons. The bias voltage positions of the corresponding intrinsic and extrinsic features are marked. Figure 2: Thermal switchover from intrinsic to defect-mediated tunnelling. Î rel ( V , T ) in the ( a ) P and ( b ) AP MTJ states within 9 K< T <80 K with d T =10 K. Consecutive curves are shifted upwards for clarity reasons. The bias voltage positions of the corresponding intrinsic and extrinsic features are marked. Full size image Thermal addressing of the F/F + ground state For T >30 K, the aforementioned intrinsic features in Î rel found for both P and AP are dominated by a new feature appearing at E = E F +1.05 eV. By comparing with the energy schematic in Fig. 1a , and by pegging E F to the band gap centre [37] (see Fig. 1a ), we attribute this feature to tunnelling across the ground state of neutral/singly charged oxygen vacancies within the barrier (that is, F/F + ). The spectral position and defect species assignment of this feature correspond quantitatively to that inferred from theoretical predictions [28] and scanning tunneling microscopy experiments [60] . We observe, however, that contrary to predictions [28] , the F/F + centre does affect transmission in the AP state, as explained hereafter. To more closely observe the impact of the F/F + level on magnetotransport, we present a separate data set of measurements in ( V , H , T ) parameter space performed on a similar MTJ. To guide the reader through the unconventional representations of our data set, we present this data set in Figs 3 , 4 , 5 . Rather than discuss all elements of a given representation and accompanying figure, we synthetically discuss the evolution of barrier heights and the TMR signal for consecutive ranges of temperature, referring to respective figures and their panels. We first present in panels of Fig. 3 Î rel data with d T =3 K in bias and temperature parameter space ( V , T ) with 5 mV and 3 K resolutions for the P and AP configurations, respectively. We then examine the corresponding thermally activated decrease in TMR by plotting (TMR( V , T )/TMR( V , T ref )−1) × 100 in Fig. 4 , where T ref =33 K in the upper panel (absolute TMR thermal decrease) and T ref = T −9 K (that is, d T =9 K) in the lower panel (relative TMR thermal decrease—plotting TMR rel =(TMR( T 2 )/TMR( T 1 )−1) × 100 with d T <9 K did not yield a useable map owing to noise issues). As a synthesis, we present the temperature-dependent evolution of the position and amplitude of the main peak of , and the relative TMR drop in Fig. 5 . To not alter or destroy our MTJs through defect-mediated electromigration [61] , we have found it necessary to limit measurements up to T =155 K at | V |=2 V, and up to T =250 K at | V |=1.3 eV. 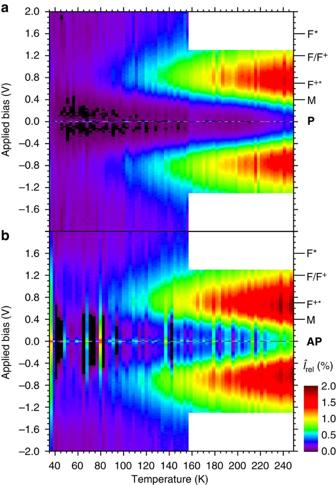Figure 3: Voltage–temperature maps of thermal impact on spin-polarized tunnelling. Îreldata in the (a) P and (b) AP MTJ states with dT=3 K within 33 K<T<252 K. Measurements above 155 K were performed only up to 1.3 V to avoid MTJ degradation/breakdown. For both panels the temperature step dT=3 K. Figure 3: Voltage–temperature maps of thermal impact on spin-polarized tunnelling. Î rel data in the ( a ) P and ( b ) AP MTJ states with d T =3 K within 33 K< T <252 K. Measurements above 155 K were performed only up to 1.3 V to avoid MTJ degradation/breakdown. 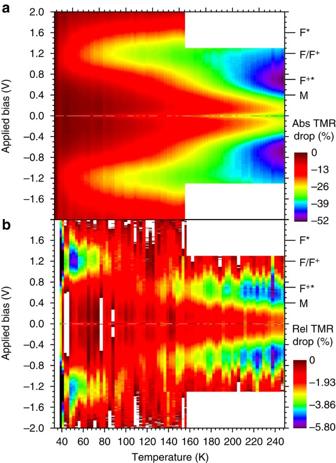Figure 4: Voltage–temperature maps of TMR thermal decrease. Impact on the spectrally resolved TMR of (a) an absolute (compared withT=33 K) and (b) a relative (9 K step) temperature increase. For both panels the temperature step d T =3 K. Full size image Figure 4: Voltage–temperature maps of TMR thermal decrease. Impact on the spectrally resolved TMR of ( a ) an absolute (compared with T =33 K) and ( b ) a relative (9 K step) temperature increase. 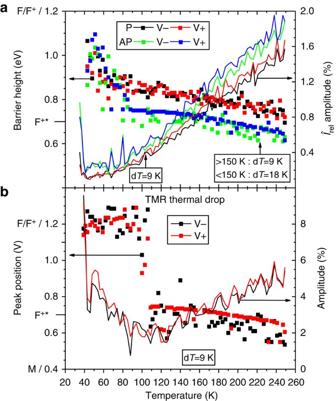Figure 5: Thermal switchover from ground to excited state-mediated tunnelling magnetotransport. Temperature dependencies of the (a) effective barrier height and amplitude of the maxima of the P and APÎrel; and of (b) the position and amplitude of the minimum in the TMR relative thermal decrease. Data for bothV>0 andV<0 are shown. Owing to very lowÎrelpeak amplitudes at low temperature and ensuing uncertainties inφ, we representφusing dT=9 K forT>150 K and dT=18 K forT<150 K. Full size image Figure 5: Thermal switchover from ground to excited state-mediated tunnelling magnetotransport. Temperature dependencies of the ( a ) effective barrier height and amplitude of the maxima of the P and AP Î rel ; and of ( b ) the position and amplitude of the minimum in the TMR relative thermal decrease. Data for both V >0 and V <0 are shown. Owing to very low Î rel peak amplitudes at low temperature and ensuing uncertainties in φ , we represent φ using d T =9 K for T >150 K and d T =18 K for T <150 K. Full size image At T =40 K, the data set in Fig. 2 clearly reveals the weight of the F/F + level on tunnelling for both P and AP MTJ configurations. Since the colour scale in Fig. 3 spans 30 K< T <250 K, the F/F + weight at T =40 K is visible in the AP data but hardly in the P data. The agreement between the two data sets nevertheless becomes apparent when considering the Î rel peak positions and amplitudes for P and AP presented in Fig. 5a . These Î rel peaks are spectrally associated with an immediate significant decrease in TMR at V =1.2 V due to thermal activation for T >30 K in both P and AP regardless of the sign of applied bias (see Figs 4 and 5b ). Thermal addressing of the F + * excited state For 30 K< T <80 K, both P and AP Î rel peaks shift rapidly from the F/F + -induced peak at 1.2 V to lower bias voltage values. Within this temperature range, the TMR thermal drop is centered at 1.2 V, but its amplitude decreases. Above 80 K, the Î rel shift lessens while the peaks’ height starts to increase markedly. Interestingly, the decrease in barrier height with increasing temperature is not the same for the P and AP channels for T >80 K. As seen in Fig. 5a , this leads to a clear difference between φ P and φ AP that we will discuss hereafter. Concurrent to this change in tunnelling barrier characteristics at T =80 K is an abrupt change in the bias position of the maximum in relative TMR thermal drop from 1.2 to 0.7 V. The amplitude of the TMR thermal drop, which was decreasing within 30 K< T <80 K, stabilizes before increasing for T >100 K. From our high-resolution ( V , T ) maps, we infer that this reflects the gradually increasing impact on magnetotransport of a feature at V ~±0.7 V. Indeed, above 80 K, this feature becomes more prominent in the TMR thermal drop, and at 100 K it totally dominates all other spectral signatures of TMR decrease. In agreement with Fig. 1a and the PL( T ) data of Fig. 1c , we explicitly ascribe this mechanism to an increase, upon thermal activation, in the weight of tunnelling across the excited state of F + centres (that is, F + *), located at E − E F =0.7 eV compared with their neutral counterparts at E − E F =−1.1 eV. Other defect states In addition to the clear spectroscopic signatures of F/F + and F + * centres within magnetotransport, we provide evidence for more subtle signatures of additional defect states. Indeed, we anticipate that centres in MgO may exhibit a 300–400-meV spectral width as schematized in Fig. 1a and in agreement with findings regarding the F + * state, as well as with the theory on the F centre [28] . Yet the spectral width at which the TMR decreases by ~−10% in the spectral vicinity of the F centre is 0.9–1.6 V at T =50 K. A similar effect occurs for Î rel (see Fig. 3 ). This doubling of spectral width, and shift to higher energies, implies the presence of an additional state at higher energy. This might reflect the excited state of F centres (that is, F*) at E = E F +1.6 eV. Referring to Supplementary Note 3 ; Supplementary Figs 5–6 , the thermal trends in I P and I AP suggest that this excited state yields a thermal onset to increased hopping transport in both P and AP channels at 70 K, as well as at 130 K. This leads to subtle onsets of TMR decreases at these temperatures. Finally, as another subtle effect, we observe a relatively resilient TMR amplitude due to thermal activation within | V |<0.4 V at T =35 K, which shrinks in spectral extent with increasing temperature and is overtaken by the contribution from the F + * state at around 100 K (see Fig. 4a ). Furthermore, we see that the spectral positions of the Î rel peaks and of the relative TMR thermal decrease may shift to values below that of the F + * state for T >200 K. Referring to Supplementary Fig. 2d , this trend is especially marked in the relative TMR thermal decrease for T >250 K. This might reflect the impact of the M ground state at 0.4 eV away from E F [25] . The aforementioned results are representative of a larger ensemble of data acquired on several samples, which we present in Supplementary Note 3 . As summarized in Table 2 , our data thus describe defect-mediated solid-state tunnelling in terms of the ground and excited states of precisely identified defect species, whose impact on magnetotransport is present at both precise values of applied bias (the ability to spectrally characterize our results for both bias polarities suggests that defects are spatially present within the barrier at least at both interfaces, if not throughout the barrier [45] ) and in specific temperature ranges. We address these two points in what follows. Table 2 Magnetotransport addressing in voltage–temperature space of select oxygen vacancy localized states. Full size table We emphasize the importance of spectrally identifying defect species within magnetotransport. Indeed, Teixeira et al. [24] , who find inelastic electron tunneling spectroscopy (IETS) signatures of defect-assisted tunnelling at precisely the same energy positions as here, remain uncertain as to why, at V =0.4 eV, there is an IETS signature in the Δ 1 -dominated P but not the Δ 5 -dominated AP channel [12] , [37] . Our data indicate that this defect does not dominate transport across our MTJs for T <250 K. Nevertheless, our work suggests that this defect is a M centre that, furthermore, is predicted [25] to promote coherent, that is, symmetry- and spin-conserved transport. Ab initio theory predicts a dominant Δ 1 symmetry for the F centre [28] . Although no such calculations exist for M centres, we argue that, owing to a similar energy position within the band gap and a rather constant Δ 1 decay parameter in this energy range [37] , this means that the M centre is dominantly of Δ 1 character, and hardly of Δ 5 character. It is thus improbable to have Δ 5 hopping conduction in the AP channel onto the M centre, especially since the M centre cannot flip [25] the carrier’s symmetry to Δ 1 for enhanced tunnelling probability off of the defect site. We thus explain the absence of an IETS signature of defect-assisted tunnelling in the AP state in certain MgO MTJs [24] . In our MTJs, however, M centres appear to dominate conduction in the AP state for T >250 K (see Supplementary Fig. 2d ). The inferred loss of coherence in magnetotransport could, in turn, explain the lower TMR that we observe at room temperature (see Table 1 ). If AP tunnelling does not proceed with respect to the M centre, it then does so with respect to the next lowest state, which in our case would be the F + * state for T >80 K. Thus, we also resolve the glaring, aforementioned contradiction between low barrier heights and enhanced TMR in MgO-based MTJs (see Table 1 ). Indeed, this shows that MgO-based MTJs with large densities of M centres benefit from a highly conductive P state, thanks to defect-assisted tunnelling with respect to a 0.4 eV barrier height defined by states that maintain the symmetry and spin polarization of charge carriers [25] , and thus conserve high values of TMR at room temperature. Experiments on such MTJs should thus yield a higher barrier height for AP than for P. In contrast to M centres, distant oxygen vacancies (that is, F/F + centres) lead to incoherent hopping transport [25] , meaning that defect-assisted tunnelling can switch the symmetry of the charge carrier. Remember that our MTJs are dominated by F-type tunnelling, while those of Teixeira et al. [24] also exhibit M-type tunnelling. Referring to our data and summary (see Table 2 ), we find that F/F + /F + */F*-assisted tunnelling leads to a relative increase in I P and I AP , with increasing temperature at the positions in the (V, T) dependence of magnetotransport expected within a picture of defect-mediated tunnelling (see Fig. 3 ) and upon correct thermal addressing of the relevant defect level. I AP < I P due to the larger decay parameter for Δ 5 states [35] , [36] , [37] , so I AP is more sensitive to a defect-induced switch from Δ 5 to Δ 1 symmetry that promotes much more efficient tunnelling transmission across the remaining thickness of MgO [37] . For T =30 K, electrons on the excited states F + * and F* decay back to the F/F + state, leading to little occupancy of these excited states compared with the ground state. Increases in MTJ conduction for both P and AP states are maximized upon correct electrical addressing of the F/F + state that is dominant at T =30 K. Within the scatter of our data, this leads for P and AP states to a similar φ . Within 30 K< T <80 K, thermal energy impedes the decay from, and thus procures increasing weight to transmission across, F + * states 0.7 eV above E F . φ , which accounts for the weight of both F/F + and F + * contributions, thus decreases monotonously, while the additional conduction channels provided by F + * levels contribute to a small increase in Î rel amplitude. Owing to scatter in our data, and perhaps to the imperfect degree of symmetry polarization of our MTJs with 200% TMR at T =30 K and V =10 mV, we cannot distinguish differences between φ P and φ AP for 30 K< T <80 K, whether in this or our other data sets (see Supplementary Note 2 ). The maximum in TMR decrease remains energetically pegged to the F/F + level, although with a decreasing amplitude as that level’s contribution to symmetry mixing saturates thermally. For T >80 K, thermal changes in the electron occupancy of F + * states (at 0.7 eV above E F ) now dominate those of the F + ground state (at 1.2 eV below E F ) (see Fig. 1 and text). Now that F + states are thermally saturated and that F + * states dominate, the decrease in φ lessens for T >80 K. Furthermore, φ AP now clearly trends to lower values than φ P with increasing T , which suggests that I AP is weighed more strongly by tunnelling with respect to the F + * level than the P channel. As discussed above, this could reflect an asymmetric relative impact on I AP and I P of opening additional conduction channels. Also, in analogy to theory on the F and F* levels [28] , if the F + and F + * levels are of different electronic character, this could alter the weight of the F + and F + * states between the Δ 1 -(Δ 5 )-dominated current in the MTJ’s P(AP) state, leading to φ AP < φ P . The F + * state is mainly responsible for promoting hopping transport in MgO [52] . This explains the renewed thermal increase, for T >80 K, in both Î rel amplitude and in the amplitude of the maximum TMR thermal decrease. Meanwhile, the bias position of the maximum in TMR thermal decrease, which tracks the thermally dominant defect level, has switched above 80 K from the F + level (at 1.2 eV) to the F + * level (at 0.7 eV). We emphasize that this trend is valid in MTJs such as ours with a dominant F/F + /F + * contribution in the P channel. Importantly, φ P > φ AP is not in contradiction with R P < R AP , but suggests that there is a competition in tunnelling probabilities with respect to localized states of defect centres and extended states of the MgO band structure [35] . Directly ascertaining the extent of this competition would require measuring Î rel up to 4 V, which is not experimentally possible without junction breakdown. Controlling the spatial position of the localized states within the tunnel barrier [27] so as to discriminate between the two tunnelling regimes could indirectly confirm this point. Also, our work reaffirms how transport in the P and AP junction states involves a different weight of Δ 1 and Δ 5 electronic symmetries. We therefore suggest that, contrary to the work of Lu et al. [21] , hopping transport in the P and AP states, which we find to be symmetry dependent, be investigated separately and at precise bias values (if the underlying theory permits it) that correspond spectroscopically to transport across identified defect centres. In conclusion, we have taken spin- and symmetry-polarized tunnelling across MgO as a canonical example of the need to take into account the electronic structure of defect sites in oxide semiconductors for advanced applications [62] , [63] , [64] . We have provided and highlighted an explicit description of thermally activated defect-assisted magnetotransport by utilizing solid-state tunnelling spectroscopy [55] to probe the ground and excited states of oxygen vacancies [49] , [52] . Spin-polarized transport across MgO-based MTJs with a ‘low’ density of M centres reproducibly proceeds with respect to F + and F + * centres for both P and AP channels, with a weighing at higher temperature (room temperature) in the AP channel towards the F + * centre compared with the P channel due to symmetry mixing. This leads, with increasing temperature, to an abrupt switchover between a F/F + -dominated TMR decrease and a F + *-dominated TMR decrease. Compared with the standard MgO MTJ theory [35] , [36] , this leads to the unexpected relation φ P > φ AP at room temperature. As future experiments on appropriate stacks [24] , [40] , [65] (and perhaps those of ref. 43 with high TMR) with possible defect control [27] can now explicitly confirm, we expect that a sufficient density of M centres would lower φ P to that centre’s energy position of ~0.4 eV from E F (see Table 1 ), thereby yielding φ P < φ AP and larger values of TMR. This shows how the effective barrier height of a MTJ reflects the energy position of all defects within the barrier dielectric relative to E F , as weighed by the thermal activation of a given defect species within a precise temperature range. We thus resolve the contradiction between low barrier heights and large values of TMR in MgO MTJs. In the process, we provide a very important nuance to the generally accepted, intuitive paradigm [20] , [27] , [28] that reducing defect densities will lead to improved TMR ratios. Indeed, as predicted theoretically [25] , certain defect species in MgO (that is, M centres) can actually promote resilient magnetotransport under thermal excitation, while others (that is, F/F + ) promote a thermally induced TMR decrease due to a more efficient, defect-induced mixing of electronic symmetries. To help clarify the varying results in the literature (see Table 1 ), we thus call on the MgO magnetotransport community to systematically report RA products, P and AP barrier heights for key temperatures corresponding to the thermal activation of precise defects using the physical technique of Î rel rather than simple geometrical tunnelling models, such as Simmons and Brinkman that cannot account for multiple barrier energy levels (see Supplementary Note 4 ; Supplementary Table 2 ). In this spirit, we can thus ascribe local transport on the electrical hotspot and background of MgO barriers that are sputter-grown with 0% (10%) oxygen in the argon plasma [27] to M and F/F + (F/F + and conduction or VB edges) centres. Electrical noise [26] , [66] and memristance [32] , [34] studies across MgO-based MTJs can immediately benefit from the clarified defect-mediated tunnelling potential landscape that we propose here. Research groups that can smoothly vary the MgO barrier thickness across a series of MTJs (for example, ref. 40 ) could, by exploring RA products in ( V , T ) parameter space, (1) obtain a defect-resolved mapping of the tunnelling attenuation parameter to be compared with theory [28] ; and (2) identify how the thickness dependence may implicate varying defect species. MgO-based spin-torque nano-oscillators [16] rely precisely on defect-mediated low barrier heights to achieve critical current densities, which should motivate additional tunnelling transmission theory [25] , [28] across M and F + * states that lie close to E F . More generally, oxide-based memristance studies [67] could strongly progress if the electronic structure of the defects that underscore memristive activity was explicitly considered. Finally, we recommend considering magnetotransport results across more exotic oxides such as ferroelectrics [3] and multiferroics [4] from the presently outlined perspective of defect-assisted transport. Ta(5)/Co(10)/IrMn(7.5)/FeCoB(4)/MgO(2.5)/FeCoB(4.5)/Ta(5)/Pt(5) samples were sputter-grown at the Institute Jean Lamour (Nancy) on Corning 1737 glass substrates [68] . MgO was sputtered in a pure Ar partial pressure. All numbers are in nanometres. Stacks were post-annealed in an in-plane magnetic field of 200 Oe for 1 h at 300 °C to both crystallize the MgO barrier and pin the lower electrode, thanks to the IrMn antiferromagnetic layer. Samples were then processed within the STNano technological platform by optical lithography into arrays of junctions with sizes varying between 14 and 40 μm in diameter [8] . Typical resistance-area values are 6 × 10 7 Ω μm 2 (see Supplementary Note 3 for a RA map). SiO 2 (150 nm) was used as the passivation layer, and the electrical contact was provided by the Al (40 nm)/Au (40 nm) bilayer. The magnetotransport data of Fig. 2 and Supplementary Fig. 4 were acquired on a liquid He flow bench with a base T =9 K, while those of Fig. 3 and Supplementary Figs 2–3 were acquired on a cryo-free bench with a base T =33 K. In the former bench, a helium-sample environment guarantees thermal accuracy between the sample and nearest thermal sensor. In the latter bench, a Cernox diode was mounted on the sample holder so as to measure the test sample temperature for all nominally requested temperatures. Optical experiments were performed on a similar structure as the one presented above, but devoid of the top metal stack. How to cite this article: Schleicher, F. et al. Localized states in advanced dielectrics from the vantage of spin- and symmetry-polarized tunnelling across MgO. Nat. Commun. 5:4547 doi: 10.1038/ncomms5547 (2014).